The impact of nitrogen oxides on electrochemical carbon dioxide reduction The electroreduction of carbon dioxide offers a promising avenue to produce valuable fuels and chemicals using greenhouse gas carbon dioxide as the carbon feedstock. Because industrial carbon dioxide point sources often contain numerous contaminants, such as nitrogen oxides, understanding the potential impact of contaminants on carbon dioxide electrolysis is crucial for practical applications. Herein, we investigate the impact of various nitrogen oxides, including nitric oxide, nitrogen dioxide, and nitrous oxide, on carbon dioxide electroreduction on three model electrocatalysts (i.e., copper, silver, and tin). We demonstrate that the presence of nitrogen oxides (up to 0.83%) in the carbon dioxide feed leads to a considerable Faradaic efficiency loss in carbon dioxide electroreduction, which is caused by the preferential electroreduction of nitrogen oxides over carbon dioxide. The primary products of nitrogen oxides electroreduction include nitrous oxide, nitrogen, hydroxylamine, and ammonia. Despite the loss in Faradaic efficiency, the electrocatalysts exhibit similar carbon dioxide reduction performances once a pure carbon dioxide feed is restored, indicating a negligible long-term impact of nitrogen oxides on the catalytic properties of the model catalysts. The electrochemical CO 2 reduction (CO 2 RR) provides a promising, sustainable avenue to generate value-added fuels and chemicals from greenhouse gas CO 2 [1] , [2] . Depending on the choice of electrocatalyst, CO 2 can be converted into a variety of single-carbon (C 1 ; e.g., carbon monoxide, formic acid, methanol, and methane) and multi-carbon (C 2+ ; e.g., ethylene, ethanol, acetate, and n-propanol) products with tremendous market potentials [3] , [4] , [5] , [6] , [7] , [8] . While CO 2 RR is being actively studied, most studies are conducted using highly pure CO 2 feed [9] , [10] . For commercial applications, the most commonly available CO 2 sources are industrial point sources, such as chemical and power plants; [11] however, CO 2 gas emitted from these sources often contain a variety of contaminants, such as sulfur oxides (SO x ), nitrogen oxides (NO x ), O 2 , and volatile organic compounds (VOC) (Fig. 1a ) [12] , [13] , [14] . Therefore, there is an urgent need to understand the potential impact of common contaminants in industrial CO 2 sources on the catalyst properties in CO 2 RR. Fig. 1: CO 2 electrolysis technology using industrial CO 2 point sources. ( a ) Schematics of CO 2 electrolysis with CO 2 stream obtained from point sources containing impurities such as nitrogen oxides (NO x ), sulfur oxides (SO x ), O 2 , and volatile organic compounds (VOC) and potential influence of impurities in CO 2 electroreduction (CO 2 RR). ( b ) Standard potential vs. reversible hydrogen electrode (RHE) for CO 2 RR, hydrogen evolution reaction (HER), NO 2 reduction (NO 2 RR), NO reduction (NORR), and N 2 O reduction (N 2 ORR). 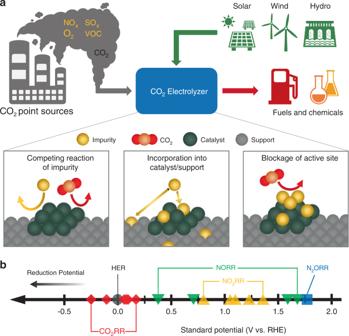Fig. 1: CO2electrolysis technology using industrial CO2point sources. (a) Schematics of CO2electrolysis with CO2stream obtained from point sources containing impurities such as nitrogen oxides (NOx), sulfur oxides (SOx), O2, and volatile organic compounds (VOC) and potential influence of impurities in CO2electroreduction (CO2RR). (b) Standard potential vs. reversible hydrogen electrode (RHE) for CO2RR, hydrogen evolution reaction (HER), NO2reduction (NO2RR), NO reduction (NORR), and N2O reduction (N2ORR). Detailed reactions are provided in Supplementary Table1. Detailed reactions are provided in Supplementary Table 1 . Full size image Gas impurity in CO 2 can affect the performance of CO 2 RR electrocatalysts as we demonstrated in the case of SO 2 [15] , where a trace amount of SO 2 in the feed is sufficient to alter the product selectivity of Cu catalyst substantially. The potential impacts of impurity include lowering Faradaic efficiency (FE; i.e., number of electrons transferred to desired products divided by the total number of electrons passed in the system) due to competing reactions of impurity over CO 2 , altering the property of the catalyst by incorporating into the catalyst and/or support, and adsorbing on the catalyst surface to physically block the active sites (Fig. 1a ). To date, there are only a few studies focusing on understanding how the presence of contaminants influences the behavior of electrocatalysts under CO 2 RR conditions [15] , [16] , [17] , [18] , [19] , [20] , [21] . For example, NO x is one of the major contaminants present in industrial CO 2 point sources with a typical concentration of 1000 ppm [12] , [13] , [14] . The NO x contaminants typically consist of 90–95% nitric oxide (NO) and 5–10% nitrogen dioxide (NO 2 ) [22] . Additionally, nitrous oxide (N 2 O) is also a common byproduct formed in the NO x removal process [23] , which has a relatively low reactivity in comparison to other NO x . A previous study has shown that 200 ppm of NO has a negligible influence on Cu catalysts in CO 2 RR in a conventional batch cell [18] . Furthermore, less than or equal to 1667 ppm of NO 2 has shown to be either beneficial or neutral, and greater than 1667 ppm of NO 2 has shown to be detrimental in CO 2 RR, mainly due to a reduction in pH of the electrolyte, also on Cu catalysts in a conventional batch cell [19] . 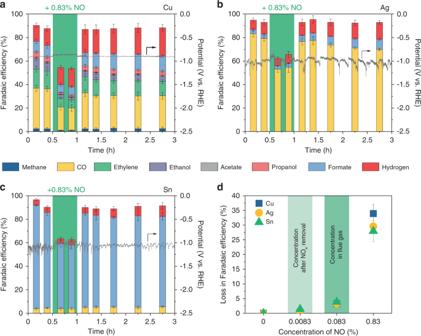Fig. 2: CO2electroreduction performance in the presence of NO. Faradaic efficiency and applied potential vs. time on (a) Cu, (b) Ag, and (c) Sn catalysts at a constant current density of 100 mA cm−2in 1 M KHCO3for 3 h. Gas feeds were 83.3% CO2and 16.7% Ar, and 83.3% CO2, 15.87% Ar, and 0.83% NO (green). 0.83% NO was introduced at 0.5 h for 0.5 h. Corresponding Faradaic efficiencies are provided in Supplementary Tables2–4. (d) Effect of different concentrations of NO in CO2electroreduction on Cu, Ag, and Sn catalysts. 0.083% and 0.0083% represent the typical NOxconcentrations in flue gases and flue gases after NOxremoval processes, respectively. Corresponding Faradaic efficiencies are provided in Supplementary Table6. Error bars represent the standard deviation of three independent measurements. However, the behavior of various NO x impurities in CO 2 RR at industrially relevant high current densities (>100 mA cm −2 ) has not been explored yet. In this work, we investigate the influence of NO x (i.e., NO, NO 2 , and N 2 O) in CO 2 RR using a three-compartment flow cell. Three model electrocatalysts, including copper (Cu), silver (Ag), and tin (Sn), are selected to represent the most studied catalysts for C 2+ products, carbon monoxide (CO), and formate, respectively. Most NO x contaminants in the CO 2 feed significantly reduce the CO 2 RR FE because the electrochemical reduction of NO x occurs at much more positive potentials than CO 2 RR (Fig. 1b ). NO and NO 2 impurities have more severe impacts on CO 2 RR FE than N 2 O, likely due to the greater number of electrons required in the NO x reactions. Despite the loss of CO 2 RR FE, none of the three catalysts exhibits a significant change of product selectivity after removing the NO x impurity from the CO 2 feed. Moreover, we employ gas chromatography (GC), spectrophotometry, and flow electrochemical mass spectrometry (FEMS) to analyze the products of electroreduction of NO, the dominant component of NO x in industrial point sources, in which the major products are ammonia (NH 3 ), hydroxylamine (NH 2 OH), N 2 , and N 2 O. Investigation of the effect of different concentrations of NO in CO 2 RR shows that NO x at typical concentrations in flue gases is compatible with CO 2 RR. 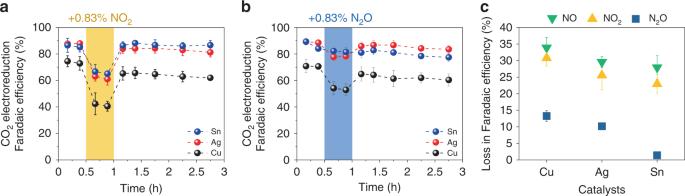Fig. 3: CO2electroreduction performance in the presence of NO2and N2O. CO2electroreduction Faradaic efficiency, excluding hydrogen Faradaic efficiency, vs. time with the introduction of (a) 0.83% NO2(yellow) and (b) 0.83% N2O (blue) on Cu, Ag, and Sn catalysts at a constant current density of 100 mA cm−2in 1 M KHCO3for 3 h. Gas feeds were 83.3% CO2and 16.7% Ar, and 83.3% CO2and 15.87% Ar with 0.83% NO2or 0.83% N2O. NO2and N2O were introduced att= 0.5 h for 0.5 h. Corresponding Faradaic efficiencies are provided in Supplementary Figs.6and7, and Supplementary Tables7–12. (c) Loss in Faradaic efficiency during CO2electroreduction from the introduction of 0.83% NO, 0.83% NO2, and 0.83% N2O on Cu, Ag, and Sn catalysts. Corresponding Faradaic efficiencies are provided in Supplementary Table13. Error bars represent the standard deviation of three independent measurements. Electrodes were prepared by loading commercial Cu, Ag, and Sn particles on a gas diffusion layer (GDL), a microporous carbon paper which provides mechanical support, electrical conductivity, and hydrophobicity. Scanning electron microscopy (SEM) images of the as-prepared electrodes confirm a uniform deposition of metal nanoparticles on GDL, covering the majority of the GDL surface (Supplementary Fig. 1 ). Electrochemical experiment was performed in a three-compartment flow cell, in which CO 2 gas is directly fed to the electrode-electrolyte interface, enabling CO 2 RR at high current densities (Supplementary Fig. 2 ). NO x impurities were mixed with CO 2 gas feed prior to entering the flow cell. As the concentration of NO x in typical exhaust streams may be as high as ~3,000 ppm (i.e., 0.3 vol. %) [13] , conservative streams of 83.3% CO 2 , 15.87% Ar, and 0.83% NO x were used for most studies. To keep the CO 2 partial pressure constant during the introduction of NO x , which contains Ar, CO 2 partial pressure was maintained at 0.833 bar throughout the study by using a mixture of 83.3% CO 2 and 16.7% Ar when NO x was not introduced. Impact of NO x impurities on CO 2 electroreduction The influence of NO in CO 2 RR on Cu, Ag, and Sn catalysts was first evaluated at a constant current density of 100 mA cm −2 (Fig. 2a–c ). The CO 2 RR experiment was performed by switching the gas feed from 83.3% CO 2 and 16.7% Ar (0–0.5 h) to 83.3% CO 2, 15.87% Ar, and 0.83% NO (green region; 0.5–1 h) and back to 83.3% CO 2 and 16.7% Ar (1–3 h). With 83.3% CO 2 and 16.7% Ar, before exposure to NO, Cu catalyst produced a wide range of C 1 (i.e., methane, CO, and formate) and C 2+ (i.e., ethylene, ethanol, acetate, and propanol) products. In the cases of Ag and Sn catalysts, the major products were CO and formate, respectively. The observed CO 2 RR selectivity of the Cu, Ag, and Sn catalysts was consistent with the previous reports [6] , [7] . Fig. 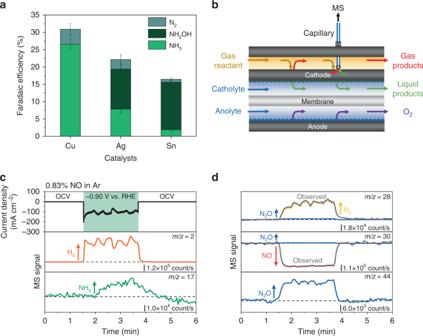Fig. 4: Investigation of the NO electroreduction products. (a) Faradaic efficiency of NO electroreduction products produced during electrolysis with 83.3% CO2, 15.87% Ar, and 0.83% NO on Cu, Ag, and Sn catalysts at a constant current density of 100 mA cm−2in 1 M KHCO3for 3 h. Corresponding Faradaic efficiencies are provided in Supplementary Table14. Error bars represent the standard deviation of three independent measurements. (b) Schematic of flow electrochemical mass spectrometry (FEMS) setup. (c) Measured current density vs. time, and deconvoluted MS signal vs. time form/z= 2,m/z= 17,(d)m/z= 28,m/z= 30, andm/z= 44 from FEMS on Cu catalyst in 1 M KHCO3with 0.83% NO in Ar. −0.90 V vs. RHE was applied for approximately 2 min starting att= 1.5 min. NORR products have been deconvoluted using the mass spectra of individual products shown in Supplementary Fig.17. Additional information is provided in the Methods section and Supplementary Figs.18and19. 2: CO 2 electroreduction performance in the presence of NO. Faradaic efficiency and applied potential vs. time on ( a ) Cu, ( b ) Ag, and ( c ) Sn catalysts at a constant current density of 100 mA cm −2 in 1 M KHCO 3 for 3 h. Gas feeds were 83.3% CO 2 and 16.7% Ar, and 83.3% CO 2 , 15.87% Ar, and 0.83% NO (green). 0.83% NO was introduced at 0.5 h for 0.5 h. Corresponding Faradaic efficiencies are provided in Supplementary Tables 2 – 4 . ( d ) Effect of different concentrations of NO in CO 2 electroreduction on Cu, Ag, and Sn catalysts. 0.083% and 0.0083% represent the typical NO x concentrations in flue gases and flue gases after NO x removal processes, respectively. Corresponding Faradaic efficiencies are provided in Supplementary Table 6 . Error bars represent the standard deviation of three independent measurements. Full size image When 0.83% NO was introduced at t = 0.5 h, the total CO 2 RR FE decreased noticeably on all three catalysts (Fig. 2a–c ). On average, the losses in CO 2 RR FE accounted for 33.9, 29.6, and 27.9% on Cu, Ag, and Sn, respectively (Fig. 2d ), which is likely due to the preferential reduction of NO over CO 2 . 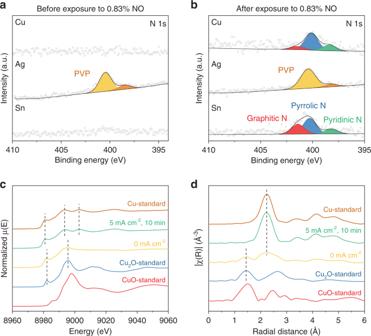Fig. 5: Evaluation of the influence of NO on the catalyst structure. XPS measurements of Cu, Ag, and Sn electrodes (a) before (t= 0 h) and (b) after exposure to 0.83% NO (t= 1 h) during CO2electrolysis. Corresponding XPS data is provided in Supplementary Fig.27and Supplementary Table15. Cu K-edge (c) XANES and (d) EXAFS spectra of spent Cu catalyst after exposure to 0.83% NO during CO2electrolysis. Cu foil, Cu2O, and CuO were used as references. Assuming NO is fully converted to NH 3 , conversions of NO during CO 2 RR are between 48% and 60% (Supplementary Table 5 ). As shown in Fig. 1b , the standard potentials of NORR are much more positive than those of CO 2 RR. For instance, the standard potential of NORR to N 2 is 1.68 V vs. RHE, while the standard potentials of CO 2 RR are between −0.250 and 0.169 V vs. RHE. Cyclic voltammetry (CV) measurements under CO 2 with 0.83% NO also confirmed that NORR is more favorable than CO 2 RR on Cu, Ag, and Sn catalysts (Supplementary Fig. 3 ). On all three catalysts, onset potentials and cathodic currents shifted to more positive potentials when 0.83% NO was introduced to the CO 2 stream. CV measurements under different concentrations of NO in Ar also confirmed more positive onset potentials of NORR than CO 2 RR and showed that NORR at 0.83% NO is mass transport limited (Supplementary Fig. 4 ). After restoring 83.3% CO 2 and 16.7% Ar, the CO 2 RR performance and the total CO 2 RR FE on all three catalysts quickly recovered and were stable for additional 2 h of electrolysis. No obvious change in selectivity was observed for any of the three catalysts, suggesting that the exposure to NO did not alter the catalyst property in any significant way. There is a slight increase in H 2 FE over time (Fig. 2a–c ), but it is likely due to the slow flooding of the electrode (Supplementary Fig. 5 ) [24] . To obtain insight on the influence of NO x in CO 2 RR at typical concentrations of NO x in point sources, we evaluated the effect of 0.083% and 0.0083% NO, representing the typical NO x concentrations in flue gases and flue gases after NO x removal processes [22] , respectively, in CO 2 RR (Fig. 2d ). Although the losses in FE at 0.83% NO were detrimental, the effect of NO was less severe at 0.083%, with less than 5% losses in FE, and negligible at 0.0083% NO. Therefore, NO at typical concentrations of NO x in flue gases is compatible with CO 2 RR, although complete removal of NO x is desired to maximize CO 2 RR FE. NO 2 is another major contaminant in industrial CO 2 point sources (5–10% of NO x ), and a substantial amount of N 2 O may also be formed as a byproduct during the NO x removal process [22] , [23] . Thus, we further investigated the influence of NO 2 and N 2 O in CO 2 RR on Cu, Ag, and Sn catalysts following the similar experimental procedure to the NO experiment. When 0.83% NO 2 was introduced at t = 0.5 h (yellow region), the CO 2 RR FE decreased on all three catalysts (Fig. 3a ). The decrease in the total FEs were 30.8, 25.6, and 22.9% on Cu, Ag, and Sn catalysts, respectively. Similarly, when 0.83% N 2 O was introduced (blue region), the total CO 2 RR FE decreased by 11.4, 10.2, and 1.4% on Cu, Ag, and Sn catalysts, respectively (Fig. 3b ). Distinct from Cu and Ag catalysts, Sn catalyst did not show a significant loss of the CO 2 RR FE in the presence of N 2 O, which is likely due to the poor activity of Sn for N 2 ORR [25] . Sn catalyst maintained a high CO 2 RR FE over the course of 3 h of electrolysis, suggesting the resistive feature of Sn catalyst to N 2 O impurity. As shown in Fig. 1b , standard potentials of NO 2 and N 2 O are also more positive than those of CO 2 RR, and therefore, we attribute the loss of the CO 2 RR FE to the preferential reduction of NO 2 and N 2 O over CO 2 , which is further supported by the CV study (Supplementary Figs. 8 – 11 ). When a pure CO 2 feed was restored, the total CO 2 RR FE on all three catalysts quickly recovered, suggesting that the exposure of NO 2 and N 2 O does not affect the property of the catalysts. Fig. 3: CO 2 electroreduction performance in the presence of NO 2 and N 2 O. CO 2 electroreduction Faradaic efficiency, excluding hydrogen Faradaic efficiency, vs. time with the introduction of ( a ) 0.83% NO 2 (yellow) and ( b ) 0.83% N 2 O (blue) on Cu, Ag, and Sn catalysts at a constant current density of 100 mA cm −2 in 1 M KHCO 3 for 3 h. Gas feeds were 83.3% CO 2 and 16.7% Ar, and 83.3% CO 2 and 15.87% Ar with 0.83% NO 2 or 0.83% N 2 O. NO 2 and N 2 O were introduced at t = 0.5 h for 0.5 h. Corresponding Faradaic efficiencies are provided in Supplementary Figs. 6 and 7 , and Supplementary Tables 7 – 12 . ( c ) Loss in Faradaic efficiency during CO 2 electroreduction from the introduction of 0.83% NO, 0.83% NO 2 , and 0.83% N 2 O on Cu, Ag, and Sn catalysts. Corresponding Faradaic efficiencies are provided in Supplementary Table 13 . Error bars represent the standard deviation of three independent measurements. Full size image A comparison of the losses in FE due to the various NO x impurities is presented in Fig. 3c . NO and NO 2 show greater losses in FE than N 2 O on all three catalysts, likely due to the greater number of electrons required in the reactions. As will be discussed in the following section, the main products of NORR are NH 3 and NH 2 OH, which require 5 and 3 electrons, respectively, while the main product of N 2 ORR is N 2 , which only requires 2 electrons. Given that all NO x readily reacts at the catalyst surface, the same amount of NO and NO 2 consume more electrons than N 2 O, causing greater losses in CO 2 RR FE. Among all the catalysts, the Cu catalyst suffers the largest FE loss on all NO x impurities, followed by Ag and Sn catalysts. Indeed, Cu has been demonstrated as one of the more active metals for the electroreduction of NO [26] and N 2 O [25] , in which Cu achieved high FE in N 2 ORR to N 2 at relatively low overpotentials. The results suggest that Cu is an effective electrocatalyst for NO x reduction, which may be further explored in future studies. Furthermore, pH was measured at the outlet of the electrolyzer at different time points (i.e., before, during, and after NO x introduction) to investigate the effect of NO x on the electrolyte pH (Supplementary Fig. 12 ). The measured pH shows that the presence of NO and N 2 O has a negligible effect on the pH, while the presence of NO 2 slightly decreases the pH by 0.03. Although NO 2 hydrolyzes to produce nitric acid and nitrous acid [27] , the effect in pH is very small, possibly due to the small amount of NO 2 in the gas feed, rapid reaction of NO 2 at the catalyst surface which prevents NO 2 from penetrating to the bulk electrolyte, and a flowing electrolyte which is constantly replenished. Identification of NO x reduction products The electrochemical reduction products of NO, the major component of NO x in industrial point sources, were further investigated. As NH 3 , NH 2 OH, N 2 , and N 2 O have been suggested as the main products in NORR [26] , [28] , [29] , NH 3 and NH 2 OH were detected via spectrophotometry (Supplementary Figs. 13 and 14 ), and N 2 was detected via GC (Supplementary Fig. 15 ). We note that the concentration of N 2 O in the gas product stream was below the detection limit of GC, suggesting that N 2 O FE was below 2% FE on all three catalysts. As shown in Fig. 4a , NORR product selectivity varied among different catalysts. Cu primarily produced NH 3 and N 2 , with no NH 2 OH, Ag produced a mixture of NORR products, and Sn primarily produced NH 2 OH. These observations are consistent with previous reports, in which Cu has been demonstrated as an effective catalyst for NORR to NH 3 [26] , and Sn has been used as a dopant in Pt to shift the selectivity from NH 3 to NH 2 OH in nitrate reduction [30] . Fig. 4: Investigation of the NO electroreduction products. ( a ) Faradaic efficiency of NO electroreduction products produced during electrolysis with 83.3% CO 2 , 15.87% Ar, and 0.83% NO on Cu, Ag, and Sn catalysts at a constant current density of 100 mA cm −2 in 1 M KHCO 3 for 3 h. Corresponding Faradaic efficiencies are provided in Supplementary Table 14 . Error bars represent the standard deviation of three independent measurements. ( b ) Schematic of flow electrochemical mass spectrometry (FEMS) setup. ( c ) Measured current density vs. time, and deconvoluted MS signal vs. time for m/z = 2, m/z = 17, (d ) m/z = 28, m/z = 30, and m/z = 44 from FEMS on Cu catalyst in 1 M KHCO 3 with 0.83% NO in Ar. −0.90 V vs. RHE was applied for approximately 2 min starting at t = 1.5 min. NORR products have been deconvoluted using the mass spectra of individual products shown in Supplementary Fig. 17 . Additional information is provided in the Methods section and Supplementary Figs. 18 and 19 . Full size image To further probe the formation of NORR products with greater sensitivity and determine the formation of N 2 O, we employed the FEMS (Fig. 4b and Supplementary Fig. 16 ), which allows us to continuously measure gas and volatile liquid products operando with a low detection limit and a short response time by continuously pulling products to the mass spectrometry (MS) near the surface of the electrodes (See Methods for more details). The MS probe was placed near the working electrode from the gas channel side, and the MS signals linked to possible products were tracked over time. We conducted the FEMS measurement on the Cu catalyst using 0.83% NO in Ar (in the absence of CO 2 ), because the ionization of N 2 ( m/z = 28, 14) and N 2 O ( m/z = 44, 30, 28, 14) produces the same fragments with CO 2 and various CO 2 reduction products [31] , [32] , [33] , complicating the reliable analysis of the NORR products (see Supplementary Note for more details). MS signals of the FEMS measurement under a continuous feed of 0.83% NO are presented in Fig. 4c, d . When a constant potential of −0.90 V vs. RHE was applied at t = 1.5 for ~2 min, MS signals of NO ( m/z = 30) decreased while those of H 2 ( m/z = 2), NH 3 ( m/z = 17), N 2 ( m/z = 28) and N 2 O ( m/z = 44) increased (Fig. 4c, d ), indicating the consumption of NO and the formation of H 2 , NH 3 , N 2 , and N 2 O. The formation of NH 3 and N 2 detected by FEMS is in agreement with the results obtained from spectrophotometry and GC analysis, respectively. The production of N 2 O, which was difficult to measure via GC, was clearly observed in FEMS, suggesting that N 2 O is one of the NORR products. NH 2 OH was not detected in FEMS, because it is nonvolatile [30] . Similarly, FEMS results also suggest the formation of N 2 and N 2 O on Ag and Sn catalysts (Supplementary Figs. 20 – 25 ). However, the formation of NH 3 was observed only on Ag and not on Sn, likely due to the small amount of NH 3 produced on Sn. Collectively, NH 3 , NH 2 OH, N 2 , and N 2 O have been determined as the NORR products. The analysis of the NORR products further confirms that the loss in CO 2 RR FE is due to the preferential reduction of NO over CO 2 . In the case of N 2 ORR, a substantial amount of N 2 was quantified with a GC (Supplementary Fig. 26 ). While the losses of CO 2 RR FE were 11.4%, 10.2%, and 1.4% on Cu, Ag, and Sn catalysts, respectively, the amounts of N 2 detected were 8.2%, 7.3%, and 0.5% of the total FE, respectively, accounting for the majority of the loss in the CO 2 RR FE. Small amount of N 2 detected on Sn catalyst demonstrates the resistive nature of Sn catalyst in N 2 ORR. Characterization of catalyst structures in the presence of NO x X-ray photoelectron spectroscopy (XPS) measurements were conducted to reveal the influence of NO x on the surface electronic structure and the chemical environment of the catalysts. The samples were obtained at various points of the CO 2 RR experiment, including before exposure to NO x , after exposure to NO x , and at the end of 3-h electrolysis. As shown in Fig. 5a , the Cu and Sn electrodes before the exposure to NO x did not show any noticeable peak in N 1 s XPS measurements. In contrast, Ag showed two distinct peaks at 400.5 eV and 398.5 eV, which can be attributed to polyvinylpyrrolidone (PVP) [34] , [35] , a surfactant used in the nanoparticle synthesis. The XPS measurements obtained after the NO exposure ( t = 1 h) exhibited new N 1 s peaks on Cu and Sn electrodes (Fig. 5b ). The peaks at 401.4 eV, 400.2 eV, and 398.2 eV can be assigned to graphitic, pyrrolic, and pyridinic N, respectively [36] , [37] , suggesting that incorporated N atoms mainly interact with carbon in GDL rather than metal catalysts (metal nitride peaks typically observed near 397 eV) [38] , [39] . The XPS measurements obtained after 3-h electrolysis show that the N incorporated in the electrode surface was still intact after additional 2 h of CO 2 RR (Supplementary Fig. 27 and Supplementary Table 15 ), with the total amount of N in the Cu and Sn electrodes remaining relatively unchanged. In the cases of 0.83% NO 2 and 0.83% N 2 O, the XPS measurements show similar N incorporation in GDL (Supplementary Figs. 28 and 29 , and Supplementary Tables 16 and 17 ). Regarding the Ag electrode, the XPS investigation of N incorporation associated with NO x was largely limited by the presence of the PVP surfactant. Fig. 5: Evaluation of the influence of NO on the catalyst structure. XPS measurements of Cu, Ag, and Sn electrodes ( a ) before ( t = 0 h) and ( b ) after exposure to 0.83% NO ( t = 1 h) during CO 2 electrolysis. Corresponding XPS data is provided in Supplementary Fig. 27 and Supplementary Table 15 . Cu K-edge ( c ) XANES and ( d ) EXAFS spectra of spent Cu catalyst after exposure to 0.83% NO during CO 2 electrolysis. Cu foil, Cu 2 O, and CuO were used as references. Full size image To further confirm the incorporation of N into GDL rather than the formation of metal nitrides, we increased the catalyst loading to 2.0 mg cm −2 , which created a thick layer of catalyst on the GDL with much less exposure of GDL in the XPS measurement. After exposure to 0.83% NO during CO 2 electrolysis, the N 1 s signal was not detected on the Cu and Sn electrodes with the increased catalyst loading, whereas the XPS measurements for the Ag electrode clearly shows the N 1 s signal, which is due to the presence of PVP on the surface of Ag catalyst (Supplementary Fig. 30 ). Conversely, when the same experiment was repeated with GDL without any catalyst, N species was still detected, confirming the incorporation of N into GDL (Supplementary Fig. 30 ). Experiments using NO 2 and N 2 O show similar incorporation of N into GDL (Supplementary Fig. 30 ). To probe the influence of NO x impurity on the oxidation state of the Cu catalyst, we conducted X-ray absorption spectroscopy (XAS) measurements using a customized XAS batch cell (Supplementary Fig. 31 ). Because of the toxicity of the NO x gases, we did not use the NO x gases directly at the synchrotron X-ray beamline but conducted XAS experiments with the electrodes taken out of the electrolyzer at 1 h (after exposure to NO x for 0.5 h) during CO 2 + NO x experiments (Fig. 2a-c and Supplementary Figs. 6 and 7 ). The Cu K-edge X-ray absorption near-edge spectroscopy (XANES) spectra of the Cu catalyst after the NO exposure show a similar spectrum of the Cu 2 O standard, suggesting an average Cu oxidation state of +1 (Fig. 5c ). Extended X-ray absorption fine structure (EXAFS) result shows that the NO-exposed Cu sample contains a mixture of Cu and Cu 2 O (Fig. 5d ). Slight oxidation of Cu is likely due to the exposure of the sample in the air during sample handling. After a constant current density of 5 mA cm −2 was applied under CO 2 RR condition, the Cu catalyst was quickly reduced to metallic Cu, suggesting that a small amount of current is sufficient to fully reduce the Cu catalyst under CO 2 RR conditions. XAS measurements on Cu samples exposed to NO 2 and N 2 O also exhibited similar behaviors as the NO-treated Cu sample (Supplementary Figs. 32 and 33 ), confirming that the Cu catalyst remains or revert to fully metallic under reaction conditions after NO x is removed from the CO 2 stream. Moreover, ex-situ SEM images were obtained at various points of the experiment to evaluate the impact of NO x on the catalyst morphology. SEM images of the spent catalysts after the exposure to NO x impurities ( t = 1 h and 3 h) exhibit minimal changes in Cu and Ag catalysts (Supplementary Figs. 1 , 34 , and 35 ). Although an increase in particle size was observed in the case of Sn catalysts (Supplementary Figs. 1 and 36 ), the Sn sample obtained after 1 h of CO 2 electrolysis in the absence of NO x also showed a similar increase in particle size (Supplementary Fig. 37 ). The Sn particles likely aggregated to lower the surface energy under CO 2 RR condition regardless of NO x , and therefore, NO x impurities are not the primary cause of the size change of the Sn particles during CO 2 RR. These results suggest that the presence of NO x during CO 2 RR has a negligible impact on the catalyst morphology. In summary, we investigated the influence of various NO x (i.e., NO, NO 2 , and N 2 O) in CO 2 RR on Cu, Ag, and Sn catalysts in a flow cell. The presence of NO x impurities reduced the CO 2 RR FE due to the preferential reduction of NO x over CO 2 . The impact of NO and NO 2 is more severe than that of N 2 O in CO 2 RR due to the greater number electrons involved in NORR and NO 2 RR compared to N 2 ORR. The major NORR products are NH 3 , NH 2 OH, N 2 , and N 2 O, in which the selectivity varies among different catalysts, whereas N 2 O is primarily reduced to N 2 . Despite the loss of CO 2 RR FE, a small amount of NO x in the CO 2 feed does not alter the metallic nature of the catalyst under CO 2 RR conditions as demonstrated by the XPS and XAS measurements. Furthermore, although high concentrations of NO x may be detrimental to CO 2 RR, NO x at typical concentrations of flue gases is compatible with CO 2 RR, causing small losses in CO 2 RR FE. NO x removal process, which is a relatively mature technology, may also be employed to ensure CO 2 RR operation at maximum efficiency. This work not only demonstrates the effect of a trace amount of NO x impurities that are often present in the industrial CO 2 point sources on the most commonly studied metal catalysts, but also offers new insights on the electrochemical reduction of NO x , which has rarely been explored in the literature. Electrode preparation Commercial Cu (25 nm, Sigma-Aldrich), Ag (<100 nm, 99.5%, Sigma-Aldrich), and Sn (0.1 μm, Alfa Aesar) particles were used as cathode catalysts. Commercial IrO 2 (99.99%, Alfa Aesar) was used as an anode catalyst. The catalyst inks were prepared by dissolving 3 mg of the catalyst and 20 μl of Nafion (5 weight % in 50/50 water and isopropanol) in 3 mL of isopropanol. The catalyst ink was sonicated for at least 30 min, and 0.25 mg cm −2 of the catalyst was drop casted onto a Sigracet 29 BC GDL (Fuel Cell Store). Flow cell electrolysis The electrochemical measurements were conducted in a three-compartment flow cell with channel dimensions of 2 cm by 0.5 cm by 0.15 cm (Supplementary Fig. 2 ). The electrode area was 1 cm 2 and the distance between the electrode and the membrane was 0.15 cm. A FAA-3-hydroxide exchange membrane (Fumatech) was used to separate electrolyte in the anode and the cathode chamber. 1 M KHCO 3 was prepared by purging CO 2 (Matheson, 99.999%) into potassium carbonate (99%, Alfa Aesar) and purified using a Chelex 100 sodium salt (Sigma Aldrich). After filtering Chelex 100 sodium salt, 1 M KHCO 3 was used as an electrolyte for both catholyte and anolyte and was fed at 0.9 mL min −1 via peristaltic pumps (Cole Parmer). The total gas flow rate was maintained at 19.2 mL min −1 with different flow rates of CO 2 , Ar (Keengas, 99.999%), and NO x . For instance, 83.3% CO 2 and 16.7% Ar was prepared by flowing 16 mL min −1 CO 2 and 3.2 mL min −1 Ar via Brooks GF40 mass flow controllers. 83.3% CO 2 , 15.87% Ar, and 0.83% NO x were prepared by flowing 16 mL min −1 CO 2 with 3.2 mL min −1 of 5% NO/Ar (Matheson Gas) or 3.2 mL min −1 of 5% NO 2 /Ar (Matheson Gas) using a 50 mL gastight syringe (1050 SL, Hamilton) via a syringe pump (New Era Pump Systems). Syringes were quickly switched to another syringe before running out of gases. Similarly, 83.3% CO 2 , 15.87% Ar, and 0.83% N 2 O were prepared by flowing 16 mL min −1 CO 2 , 3.04 mL min −1 Ar, and 0.16 mL min −1 N 2 O (99.99%, Matheson Gas). N 2 O was fed by using a 10 mL gastight syringe (1010 SL, Hamilton) via a syringe pump (Cole Parmer). For NO 2 experiment, the gas outlet of the electrolyzer was connected to 2 M KOH (85%, Sigma-Aldrich) to scrub the remaining NO 2 and additional Ar was flowed at 16 mL min −1 to carry the CO 2 RR products to the GC. CV and chronopotentiometry experiments were conducted via an Autolab PG128N. For CV measurements, the electrodes were pre-reduced at 100 mA cm −2 in 83.3% CO 2 and 16.7% Ar for 10 min. The half-cell potentials were measured with respect to Ag/AgCl reference electrode (Pine Research) and calculated to the RHE scale in which E (vs. RHE) = E (vs. Ag/AgCl) + 0.209 V + 0.0591 V × pH − η IRdrop . The pH was measured at the outlet of the catholyte channel. The resistance was measured with the current-interrupt technique [40] , and the measured potential was manually post IR-corrected. Product quantification The gas products were analyzed via a multiple gas analyzer no. 5 gas chromatography system (SRI Instruments) equipped with a Molsieve 5 A and a HayeSep D column connected to a thermal conductivity detector (TCD) and a flame ionization detector (FID). Ar was used as a carrier gas with a flow rate of 19 mL min −1 and 1 mL of sample was automatically loaded to the column. The gas sample was loaded to 0.5 m HaySep D pre-column connected to 2 m Molsieve 5 A column at 0.050 min. At 0.490 min, any molecule remaining in the HaySep D precolumn was backflushed out to vent. At 2.150 min, the gas sample was automatically loaded to 2 m HaySep D column. The column temperature was maintained at 35 °C for 2.950 min, increased to 210 °C at 40 °C/min, and maintained at 210 °C until the end of the analysis. A typical GC analyses of potential CO 2 RR products, N 2 , NO, and N 2 O are provided in Supplementary Fig. 38 . 2% H 2 , 1% CO, 1% CH 4 , 1% C 2 H 4 , 0.50% C 2 H 6 , 0.25% C 3 H 6 , 0.25% C 3 H 8 in Ar (Matheson) was used to obtain the chromatogram of potential CO 2 RR products. The liquid CO 2 RR products were analyzed via 1 H nuclear magnetic resonance (NMR) with water suppression using a presaturation method (Bruker AVIII 600 MHz NMR spectrometer). The liquid sample was collected at the outlet of the electrolyzer and diluted to 25% in deionized water (DI). 500 μL of the diluted sample was mixed with 100 μL of 25 ppm (volume %) dimethyl sulfoxide (99.9%, Alfa Aesar), which was used as an internal standard, in D 2 O. NH 3 was quantified using indophenol blue method [41] with UV-vis spectroscopy (Nanodrop 2000, Thermo Scientific). 100 μL of the sample was mixed with 500 μL of alkaline hypochlorite solution (A1727, Sigma-Aldrich) and 500 μL of phenol nitroprusside solution (P6994, Sigma-Aldrich). The solution was incubated in the dark at room temperature for 20 min. 2 μL of the solution was pipetted onto the pedestal, and the absorbance was measured by UV–vis spectroscopy from 190 nm to 840 nm. The absorbance of the sample was measured at 630 nm, and the absorbance measured at 830 nm was subtracted to remove the background. The calibration curves were obtained using different concentrations of ammounium hydroxide (NH 4 OH; 28.0–30.0%, Sigma Aldrich) in 0.25 M KHCO 3 (Supplementary Fig. 13 ). NH 2 OH was quantified using a procedure modified from a procedure reported by Afkhami et al [42] . with UV–vis spectroscopy (Nanodrop 2000, Thermo Scientific). Neutral red solution was prepared by dissolving 200 mg of neutral red (Sigma-Aldrich) in 100 mL DI. Iodate solution was prepared by dissolving 1.00 g of potassium iodate (KIO 3 , 99.995%, Sigma-Aldrich) in 100 mL DI. A total of 500 μL of sample was mixed with 250 μL of 3.0 M sulfuric acid (Fisher Scientific) and 250 μL of iodate solution. After 5 min at room temperature, 500 μL of neutral red solution was added to the solution. The solution was incubated at room temperature for 20 min. In total 2 μL of the solution was pipetted onto the pedestal, and the absorbance was measured by UV–vis spectroscopy from 190 nm to 840 nm. The absorbance of the sample was measured at 510 nm, and the absorbance measured at 800 nm was subtracted to remove the background. The change in absorbance was determined by subtracting the absorbance of the sample solution from the absorbance of the solution with 0 mg L −1 NH 2 OH. The calibration curves were obtained using different concentrations of hydroxylamine (50 wt % in H 2 O, Sigma Aldrich) in 0.25 M KHCO 3 (Supplementary Fig. 14 ). Flow electrochemical mass spectrometry (FEMS) An identical flow cell with an entrance for the MS probe at the top of the gas channel was used for the FEMS measurement (Supplementary Fig. 16 ). The probe consisted of a PEEK capillary with inner diameter of 0.25 mm with PTFE membrane attached at the tip of the capillary. The PTFE membrane with a pore size of 200 μm was used to prevent the entry of aqueous electrolyte, while allowing gaseous and volatile products to enter the MS chamber. The distance between the probe and the cathode was kept constant. The electrodes were pre-reduced at 10 mA cm −2 for 5 min in Ar before the introduction of 0.83% NO. The products were detected by a Hiden Quadrupole mass spectrometer (MS). The mass fragments were detected by a secondary electron detection voltage of 1700 V with an ionization potential of 70 eV and emission current of 200 A. m/z of interest was tracked over the course of the experiment, in which a constant potential was applied for approximately 2 min starting at t = 1.5 min. For the deconvolution of m/z = 17 signal, m/z = 17 signal from the water was first determined using m/z = 18 signal. Next, the contribution from water to m/z = 17 signal was subtracted from the observed m/z = 17 signals to obtain the signal from ammonia. For the deconvolution of m/z = 28 and 44 signals, m/z = 28 and 44 signals from CO 2 in the electrolyte was first determined using m/z = 12 signal. m/z = 12 signal was smoothed using the Savitzsky-Golay method with a window of 30 data points to reduce the oscillations in the signal prior to deconvolution. Next, the contributions from CO 2 to m/z = 28 and 44 were subtracted from the observed m/z = 28 and 44 signals to obtain the signals from NORR products. m/z = 44 signal corresponded to the signal from N 2 O, and this was used to calculate the contribution of N 2 O to m/z = 28 and 30. Lastly, the contributions of N 2 O to m/z = 28 and 30 were subtracted from the m/z = 28 and 30 signals from NORR products, respectively, to yield N 2 and NO signals, respectively. All deconvolution was conducted using MATLAB. Mass spectra of NH 4 OH, NO, N 2 O, N 2 , H 2 O, and CO 2 used for the deconvolution were obtained using the same MS equipment (Supplementary Fig. 17 ). Material characterization For SEM and XPS measurements, the electrodes were first taken out of the electrolyzer after electrolysis at desired time points. The electrodes were dried in the vacuum oven (MTI Corporation) for up to three days before SEM images were acquired with Auriga 60 CrossBeam (1.5 kV). The electrodes were quickly transported to the XPS equipment (K-alpha Alpha X-ray photoelectron spectrometer system, Thermo Fisher Scientific) after drying in the vacuum oven for 5 min. The electrodes were exposed to air for less than 20 min. High-resolution XPS measurements were obtained at pass energy of 20 eV with a step size of 0.1 eV. Flood gun was turned on. Cu 2p, Ag 3d, and Sn 3d were scanned 10 times while N 1 s was scanned 30 times. Four different spots were scanned and averaged. All peaks were fitted using Thermo Avantage software with adventitious carbon referenced to the C1s peak at 284.8 eV. XAS measurement was performed at the 8-ID Beamline of the National Synchrotron Light Source II at Brookhaven National Laboratory (BNL). The electrodes were taken out of the electrolyzer at 1 h (after exposure to NO x for 0.5 h) during a 100 mA cm −1 constant current CO 2 RR experiment with the introduction of NO x (Fig. 2a–c and Supplementary Figs. 6 and 7 ). In the case of NO 2 , the samples were exposed to 0.23% NO 2 instead due to the availability of the gas at the time of the experiment. The electrodes were quickly stored in vials filled with Ar and the vials were tightly sealed with Parafilm at the home institution. The electrodes were transported to the Brookhaven National Laboratory (New York, USA) and were loaded into a XAS batch cell, which was fabricated from Teflon and 304 stainless steel, with a Kapton film window for high transmissivity for X-ray measurements (Supplementary Fig. 31 ). The electrodes were exposed to air for ~20 min before the measurement. Pt wire and Ag/AgCl were used as a counter and a reference electrode, respectively. 1 M KHCO 3 was used as an electrolyte and CO 2 was flowed at 10 mL min −1 . XAS data were analyzed using the IFEFFIT package, which included ATHENA and ARTEMIS [43] .